Pooled CRISPRi screening of the cyanobacteriumSynechocystissp PCC 6803 for enhanced industrial phenotypes Cyanobacteria are model organisms for photosynthesis and are attractive for biotechnology applications. To aid investigation of genotype-phenotype relationships in cyanobacteria, we develop an inducible CRISPRi gene repression library in Synechocystis sp. PCC 6803, where we aim to target all genes for repression. We track the growth of all library members in multiple conditions and estimate gene fitness. The library reveals several clones with increased growth rates, and these have a common upregulation of genes related to cyclic electron flow. We challenge the library with 0.1 M L-lactate and find that repression of peroxiredoxin bcp2 increases growth rate by 49%. Transforming the library into an L-lactate-secreting Synechocystis strain and sorting top lactate producers enriches clones with sgRNAs targeting nutrient assimilation, central carbon metabolism, and cyclic electron flow. In many examples, productivity can be enhanced by repression of essential genes, which are difficult to access by transposon insertion. Cyanobacteria are model organisms for photosynthetic electron flow, photorespiration, and the circadian clock [1] , [2] , [3] . In addition to their massive ecological importance, biotechnological applications of cyanobacteria have been proposed, such as microbial cell factories, where metabolism is engineered to synthesize chemicals from CO 2 using energy derived from light [4] , [5] , [6] . This widespread interest in cyanobacteria brings a need for a system-wide analysis of gene essentiality, as well as tools for elucidating gene function. Even in model cyanobacteria such as Synechocystis , approximately 45% of genes have no assigned function (Cyanobase). Historically, the transposon mutagenesis library has been used to identify loss-of-function or gain-of-function mutants in bacteria. Variants of transposon mutagenesis tag the transposon insertion site with a barcode, which enables tracking and quantification of mutant growth via next-generation sequencing (NGS). Rapid screening of libraries in multiple growth conditions is one avenue to elucidating gene function [7] . A transposon library in the cyanobacterium Synechococcus elongatus PCC 7942 (hereafter Synechococcus PCC 7942) was used to map essential genes in both constant light and diurnal growth (12 h light, 12 h dark) [8] , [9] . An alternative to transposon mutant libraries are pooled CRISPRi libraries for targeted gene repression, where unique single-guide RNA (sgRNA) genes are pooled and transformed into the strain of interest. Since the protospacer region of sgRNAs is small enough (~20 nt) to be sequenced by NGS, it can serve as a barcode and allows monitoring of the abundance of each clone in the library. Important for phenotyping, inducible CRISPRi allows modulation of essential genes. CRISPRi libraries have been applied to screen gene essentiality and diverse phenotypes in various model bacteria, including morphology, solvent tolerance, and phage resistance [10] , [11] , [12] . Inducible CRISPRi has been developed for several cyanobacteria strains [13] , [14] , but pooled sgRNA libraries have not been exploited. Here we report the construction and use of an inducible CRISPRi library of 10498 clones for the model cyanobacterium Synechocystis sp. PCC 6803 (hereafter Synechocystis ). Each clone expresses dCas9 and an sgRNA that targets a protein-coding open reading frame (ORF) or a non-coding RNA (ncRNA). We track the composition of the library during growth in multiple conditions, including different light regimes and in the presence of the organic acid L-lactate. We also screen the library for enhanced L-lactate production using droplet microfluidics (Fig. 1 ). In addition to providing fitness scores for almost all ORFs and ncRNAs in Synechocystis , our results give insights into how to engineer cyanobacteria metabolism for industrial use. We show that there are multiple gene knockdowns that increase the growth rate of Synechocystis , though these genes regulate similar processes in photosynthesis. We find far fewer diurnal-specific fitness genes in Synechocystis when compared to previously published data from Synechococcus PCC 7942. Further, we provide support for previous computational predictions that alteration of the ATP/NADPH balance can improve bioproduction in cyanobacteria. By screening both growth and productivity, this platform can yield mutants that trade biomass formation for increased productivity of a target compound. While we have focused on biotechnological traits of interest here, the CRISPRi library can be used to explore the connection between growth and robustness in many conditions, all while allowing access to modulation of essential genes. The data for all competition experiments performed with the sgRNA library can be accessed through an interactive web application [ https://m-jahn.shinyapps.io/ShinyLib/ ]. Fig. 1: Workflow for CRISPRi screening in Synechocystis . a Creating the CRISPRi library. An inducible promoter P L22 is used in Synechocystis . b The fitness or productivity of each library member is assessed by counting mutants in a bioreactor cultivation or in a sorted population using next-generation sequencing. Full size image Gene fitness during photoautotrophic growth We designed a CRISPRi library for repression of each annotated gene in Synechocystis (3546 ORFs, 1871 ncRNAs) [15] . We designed two sgRNAs for each of 3526 ORFs and 1555 ncRNAs, and one sgRNA for 20 ORFs and 316 ncRNAs, totalling 10498 sgRNAs (Methods, Supplementary Data 1 , Supplementary Data 2 ). The resulting 10498 sgRNA sequences were synthesized, pooled, and cloned into a genomic integration vector, and the pooled sgRNAs were transformed into a Synechocystis strain containing a genome-integrated, anhydrotetracycline (aTc)-inducible dCas9 cassette. The resulting Synechocystis clones were pooled and constituted the CRISPRi library. Deep sequencing of the sgRNA region of the library confirmed that all of the designed 10498 sgRNAs were present. We cultivated the library in light-limited turbidostats under two constant-light conditions, 100 μmol photons m −2 s −1 (L100) and 300 µmol photons m −2 s −1 (L300) and a light-dark diurnal condition (LD, sinusoidal illumination up to 300 µmol photons m −2 s −1 over a 12 h period followed by 12 h darkness), each with supplemented 1% CO 2 and in four replicates. Samples for NGS were taken periodically over 32 cell generations (L100 and LD cultivations were 32 days, µ ~0.03 h −1 ; L300 cultivations were 16 days, µ ~0.07 h −1 ; Supplementary Data 3 ). For each sampling point, the abundance of the 7072 sgRNAs targeting ORFs were quantified and averaged across the four replicates. The sgRNAs were grouped into five clusters based on their rate of washout (depletion) from the turbidostat (Fig. 2a ). In total, 1998 sgRNAs (28.3%) had a significant depletion in at least one condition, indicating these target genes have some contribution to cell fitness (Fig. 2b ). Cluster 1 (241 sgRNAs) contained sgRNAs that were depleted in induced and uninduced cultivations, revealing weak background leakage of dCas9 and particular sensitivity to changes in abundance of these genes. Cluster 2 (378 sgRNAs) was enriched in sgRNAs that were quickly depleted in all growth conditions. Cluster 3 (767 sgRNAs) contained sgRNAs that were more rapidly depleted in L300 than L100. Cluster 4 (612 sgRNAs) contained sgRNAs that were depleted slowly, and cluster 5 (5074 sgRNAs) contained sgRNAs that were not depleted at all. Cluster 5 combines two very similar clusters differing only in the temporary enrichment of a subset of sgRNAs, most likely due to technical variation (L300, 1 and 2 d time-points). A gene-ontology (GO term) enrichment analysis showed that clusters 1 and 2 were highly enriched for GO terms related to core cellular processes such as photosynthesis, carbon fixation, and translation (Fig. 2c ). Cyanobacteria invest most of their resources into synthesizing proteins from these groups [16] , [17] . Interestingly, nearly all sgRNAs with a low fitness score (i.e., they are depleted from the library) targeted genes whose expression were found by Jahn et al. to be regulated with growth rate (Supplementary Fig. 1 , protein abundance based on mass spectrometry measurements) [16] . Cluster 3 was enriched for a more diverse set of GO terms (e.g., secondary metabolites, cell membrane) and cluster 4 was enriched in only one GO term (nucleotide metabolism). Fig. 2: Dynamics of CRISPRi library during photoautotrophic growth. a Clustered sgRNAs by similarity of log 2 fold-change over time. Rows represent time-points sampled after induction. (L100—light with 100 µmol m −2 s −1 , L300—light with 300 µmol m −2 s −1 , LD—light-dark cycle). All log 2 fold-change values were calculated from averages of four replicate cultivations. Symbols: plus, induced, minus, non-induced, star, cluster 5 is a combination of two unchanged clusters. b Log 2 fold-change of individual sgRNAs over the course of each cultivation. Experiment run time was normalized to number of cell generations estimated from population growth rate. c Enriched gene-ontology (GO) terms for the four clusters (1–4) showing sgRNA depletion; p -value—Fisher’s exact test with elimination (see Methods). Source data are provided as a Source Data file. Full size image Fitness scores for genes in central carbon metabolism can be used to refine flux predictions of core metabolic models. Here, data revealed instances of both rigidity and plasticity in Synechocystis central carbon metabolism. For example, the production of pyruvate in Synechocystis has been predicted to be mainly through decarboxylation of oxaloacetate by NADP-dependent malic enzyme, not dephosphorylation of phosphoenolpyruvate by pyruvate kinase [18] . However, malic enzyme ( me, slr0721 ) and pyruvate kinase ( pyk2 , sll1275 ) both have low fitness scores (Supplementary Fig. 2 ). This suggests that one route to pyruvate cannot fully substitute for the loss of the other, though interpretation of pyk2 fitness is complicated by its position in an operon (see Discussion). Within the Calvin cycle, two energetically equivalent routes for synthesis of fructose-6-phosphate have been considered: through class-I fructose-bisphosphate aldolase ( fda, slr0943 ) or through transaldolase ( talB, slr1793 ) [19] . Neither of these genes had a low fitness score, though the class-II FBP/SBP aldolase gene ( cbbA, sll0018) , which is needed to synthesize sedoheptulose bisphosphate for both proposed routes, did have a low fitness score. While these results do not definitively show which route is favored under photoautotrophic conditions, they suggest that flux can operate through either route if the other is perturbed. This flexibility is in contrast to Synechococcus PCC 7942, where a transposon insertion library showed that the sole FBP aldolase gene was essential for photoautotrophic growth, and transaldolase was not [8] . We next compared fitness scores for sgRNAs in each growth condition (see Methods for calculation). Fitness scores were generally lower in the L300 condition than in L100, even when normalized to number of cell generations (Fig. 3a ). One explanation could be a higher protein turnover rate in the higher growth condition. Lower fitness scores at L300 could also be expected for genes mediating high light or redox stress acclimation. In order to find genes important for specific light conditions, we calculated gene fitness as the mean fitness of two sgRNAs, and selected only genes where both sgRNAs were present in the same cluster. We found 38 genes that were beneficial for growth in L300 but neutral in L100, according to a difference in gene fitness ≥ 3 (Fig. 3b ). This set was almost exclusively in cluster 3 and 4 and included genes related to DNA repair, proteome and redox homeostasis, and subunits of PSI and the NADPH dehydrogenase NDH-1 (Fig. 3c ). Energy dissipation and photo-stress response are thus particularly important for growth at high light. There were 22 genes with differential fitness between L100 and LD, and only 5 between L300 and LD (Supplementary Fig. 3 and 4 ). The extensive overlap between L300 and LD suggests that the LD condition may involve light stress, likely at dawn. The five genes with different fitness scores between L300 and LD include two CO 2 hydration genes ( ndh3, slr1302 ). The dearth of genes with LD-specific fitness contributions is in contrast to Synechococcus PCC 7942, where more than 100 genes were found with a transposon library to be important for LD growth [9] . This discrepancy could be attributed to the CRISPRi library comprising partial repressions and not gene knockouts. Furthermore, Synechococcus has a more pronounced day-night rhythm than Synechocystis , with a higher fraction of oscillatory transcripts and larger amplitudes [20] . Fig. 3: Genes with condition-dependent fitness in two light conditions. a Distribution of fitness score F for all sgRNAs in clusters 1–4 (color code as in Fig. 2 ). Fitness score indicates the degree of enrichment (positive) or depletion (negative) of an sgRNA, normalized to cell generations. Comparison between two light conditions (L100—light with 100 µmol m −2 s −1 and L300—light with 300 µmol m −2 s −1 ) shows sgRNAs are on average more rapidly depleted under L300 independent of number of cell generations. b Difference in fitness (Δ F ) between L100 and L300, for genes with both sgRNAs in the same cluster. Differentially depleted/enriched sgRNAs indicated in red, threshold: 3 ≤ ΔF ≤ −3. c Time courses of both sgRNAs for a selection of 18 genes with high Δ F in L100 (blue) and L300 (yellow). Source data are provided as a Source Data file. Full size image Mutants with a growth advantage Quantification of the library population over time in a turbidostat allows calculation of the maximum specific growth rate µ of each mutant (Methods). Growth-rate estimates allow for more intuitive interpretation of mutant fitness and highlights that library clones are repression mutants, not total knockouts. For example, repression of Calvin cycle genes often caused significant reduction of µ (e.g ., prk −40%, cbbA −95%), while repression of most photorespiration-related genes did not (e.g ., glcD1 −10%, glcD2 −10%; Supplementary Fig. 2 ). Many clones showed higher growth rates than the population average, notably those targeting pmgA ( mean increase for L100 and L300 + 17%) and slr1916 (mean increase + 13%). The pmgA and slr1916 repression clones also showed higher growth rates in the diurnal condition (Fig. 4a ). PmgA is a regulator involved in the high-light response in Synechocystis and a pmgA knockout mutant has an inability to reduce PSI content in high light, resulting in more efficient photosynthesis [21] . A slr1916 mutant was previously identified from a small Synechocystis transposon library on the basis of altered fluorescence kinetics and also shows a higher PSI content at high light [22] . Notably, other mutants isolated in the study of Ozaki et al. were not enriched in our library, indicating that altered PSI/PSII alone does not ensure faster growth [22] . Slr1916 was annotated based on homology as menH , an esterase in the phylloquinone pathway. However, repression of the 8 other phylloquinone pathway genes resulted in strong growth defects, suggesting slr1916 is not a key enzyme in this pathway (Supplementary Fig. 5 ). Furthermore, slr1916 is localized to the plasma membrane [23] , though its proposed substrates are soluble. Three additional sgRNA clones showed slight but significant increases in growth rate in the turbidostat data (+5%): sll1969 , an annotated triacylglycerol lipase in the same operon as pmgA; slr1340 , an uncharacterized gene encoding a predicted acetyl-transferase, and ssl2982 , encoding the non-essential ω subunit of RNA polymerase [24] . Fig. 4: Transcriptomics of faster-growing mutants. a Enrichment of faster-growing sgRNA mutants in library competition (turbidostat) experiment at L300 (300 µmol photons m −2 s −1 ), log 2 fold-change of read count over time ( n = 2 sgRNAs). b Volcano plot representation of transcriptomics data from four reconstructed sgRNA mutants. Shows log 2 fold-change for gene expression compared to the control strain (sgRNA-NT0), against adjusted p -value for each gene. Gray—non-significantly different genes, pink—significantly different genes (threshold: negative log 10 p -value ≥ 2; absolute log 2 fold-change ≥ 1). The p -value for three sgRNA mutants was outside the plotting region and was restricted to −log 10 of 50 for visibility. c Heat map representation of transcriptomics data from four reconstructed sgRNA mutants. Shows all 305 genes that were significantly different in at least one of the four mutants, clustered into two different groups based on similarity of gene expression. d Significantly different genes are sorted by Cyanobase pathways. Genes of particular interest were highlighted (see text for details). Blue and orange indicates negative and positive log 2 fold-change, respectively. Size of symbols increases with increasing absolute change. Source data underlying Fig. 4b, d are provided as a Source Data file. Full size image In an attempt to uncover common regulations among these mutants, we reconstructed axenic knockdown strains. The repression clones of pmgA , slr1916, sll1969 , and ssl2982 each had a higher maximum growth rate than the control strain, as measured in the exponential phase of batch cultivation, while the growth rate of the slr1340 repression clone was not higher than the control strain (Supplementary Fig. 6 ). We next collected transcriptomics of strains after CRISPRi induction. A pmgA clone was not included as microarray data from a pmgA knockout was reported previously [25] . From the RNA-Seq data, slr1916 and ssl2982 mutants had 143 and 248 differentially expressed genes compared to a control strain (sgRNA-NT0, with no target site in Synechocystis genome) (Fig. 4b ). A weak transcriptomic response of slr1340 and sll1969 mutants could be due to a lower repression efficiency in these clones (log 2 FC of target genes was −2.57 and −1.67, for slr1340 and sll1969 , respectively, compared to −5.37 and −4.85 for slr1916 and ssl2982 ). Clustering genes based on similarity of expression changes revealed that the same set of genes was affected for all mutants, but with stronger effects in slr1916 and ssl2982 (Fig. 4c ). The high-light responsive transcription factor RpaB ( slr0947 , regulator of phycobilisome association B) was upregulated in multiple mutants. The extensive regulon of RpaB includes likely repressor activity of linear electron transport at high light (e.g., subunits of PSII and Cyt-b 6 f), and activation activity of photoprotection and cyclic electron flow (e.g., ftsH and ssr2016 ) [26] . Other common upregulated genes are involved in electron transport ( fed7 ), and include components of the NDH-1 complex (ndhD1, ndhD2 ) and carotenoid biosynthesis ( crtQ and crtZ) (Fig. 4d ). Cyanobacterial NDH-1 complexes participate in cyclic electron flow around PSI, respiratory electron flow, and CO 2 uptake [27] . Genes that were downregulated in all four mutants were sll1851 , a small non-annotated gene, and chlN ( slr0750 ), a subunit of the light-independent operative protochlorophyllide oxidoreductase (LI-POR). Gene fitness in the presence of L-lactate The CRISPRi library is also beneficial for finding stress tolerance phenotypes, which are generally difficult to engineer rationally. The commodity chemical L-lactate has been produced in several cyanobacteria but still at relatively low titers (up to 15 mM) [28] . The tolerance of Synechocystis to L-lactate is ~0.1 M (9 g/L), at which specific growth rate is reduced by 50% (L100 condition, Supplementary Data 3 ). To identify mutants with increased tolerance to L-lactate, we cultivated the library in turbidostats with added 0.1 M sodium L-lactate (pH-adjusted) and sampled periodically for NGS (0, 16, and 32 d). We found 75 sgRNAs that were enriched during the L-lactate cultivation, but not in a NaCl control cultivation (Fig. 5a ). Eight genes were enriched with both sgRNAs (Fig. 5b ). Curiously, 19 of the enriched sgRNAs (24%) targeted genes in amino-acid metabolism and protein biosynthesis, including multiple amino-acid tRNA synthetases ( argS, aspS, asnS, glyS, gltX, metS ) (Supplementary Fig. 7 ). Many of these clones had growth defects in the absence of L-lactate (NaCl control, grey area in Supplementary Fig. 6 ), which supports the general phenomenon that slow-growing microbes are more stress tolerant [29] . Fig. 5: SgRNA clones with improved L-lactate tolerance. a Volcano plot showing enrichment of 75 sgRNAs during cultivation with added 0.1 M sodium L-lactate after 32 d, (threshold: log 2 fold-change ≥ 2, −log 10 p -value ≥ 20). Only 8 sgRNAs were enriched in a 0.1 M NaCl control cultivation. b Eight genes where both sgRNAs were enriched above average in 0.1 M L-lactate cultivation (coloured) but not NaCl cultivation (gray). Color indicates association to a cyanobase pathway. F - mean fitness score of two sgRNAs. c Mean growth rate µ (h −1 ) of selected, reconstructed knockdown strains ( n = 2 independent replicate cultivations) over the first 80 h of batch cultivation with L-lactate added to 0.1 M. Symbols show significance between the control strain (NT0) and mutants using 1-sided student’s t -test. * p -value ≤ 0.05, ** p -value ≤ 0.01 (sll1712, p = 0.019; bcp2, p = 0.006), #—only 1 replicate was used for ilvA mutant. d Example of growth advantage in batch culture with L-lactate added to 0.1 M of sgRNA clones bcp2 , aroH , and ilvA . e Absorption spectra of fastest-growing sgRNA mutants and NT0 in 0.1 M L-lactate. Arrows mark absorption maxima for pigments. CT carotenoids, PC phycocyanin, CA chlorophyll A. f Relative pigment absorption for carotenoids, phycocyanin, and chlorophyll A for the selected strains with L-lactate added to 0.1 M. Source data underlying Fig. 5a, b are provided as a Source Data file. Full size image We reconstructed nine of the repression clones to confirm growth improvement in batch cultures with added L-lactate (Fig. 5c, d , Supplementary Fig. 8 ). Of the nine clones, the sll1712 and bcp2 mutants had significantly higher growth rates than the control strain (Fig. 5c ). The bcp2 mutant (bacterioferritin co-migratory protein, a peroxiredoxin) had the largest improvement, a 49% increase in µ ( p = 0.006, student’s t -test). We tested L-lactate consumption of all mutants and found that none consumed L-lactate over a 48-hour period. The mechanism for increased tolerance in the bcp2 mutant is not known. However, thioredoxins can mediate direct reduction of cysteines on transcription factors, including the master RpaB regulator in Synechocystis [30] . The absorbance spectra of all L-lactate-tolerant mutants showed increased chlorophyll A and phycocyanin absorption in the presence of L-lactate (Fig. 5e, f ). Relative concentration of carotenoids, pigments related to the light stress response, was reduced in L-lactate tolerant mutants. We could also identify clones with growth negatively affected by L-lactate but not by NaCl (Supplementary Fig. 9 ). These targeted genes could thus be candidates for overexpression to improve tolerance. Most prominent were an antibiotic resistance gene ( zam, sll1910 ), two nucleases, the protease clpX ( sll0535 ), cytochrome M ( cytM, sll1245 ) that may act to dissipate excess electrons [31] , and sepF ( slr2073 ), an inhibitor of cell division. Screening the CRISPRi library for L-lactate productivity The CRISPRi library can be linked to screens other than growth, and we next sought to find mutant clones that had increased productivity of L-lactate. The sgRNA pool and inducible dCas9 cassette were cloned into a Synechocystis strain containing lactate dehydrogenase from Lactococcus lactis [32] . The resulting L-lactate CRISPRi library was characterized by NGS and contained 10494 unique sgRNA clones. To screen the library for a secreted product, we used droplet encapsulation and microfluidics sorting [33] , [34] . First, the L-lactate CRISPRi library was grown in shake-flasks, and gene repression was induced by addition of aTc. Cell aliquots were taken after 36 h and 66 h to assay for L-lactate productivity (Methods, Supplementary Fig. 10 ). The productivity assay involved encapsulation of cells in droplets, followed by a picoinjection of each droplet with the components of a fluorescent L-lactate assay. In each droplet, secreted L-lactate reacts with the assay, allowing droplets to be sorted based on fluorescence. The cultivation and two-time point productivity assays were done on two separate occasions, resulting in four sorting runs. For each run, approximately 180,000 cell-containing droplets were screened and 36,000 droplets were sorted. Cells could not be reliably recovered on agar plates after sorting, so we performed PCR of the sgRNA region directly from sorted droplets, followed by NGS library preparation and quantification. In each sorted sample, 1500–5000 unique clones were detected with confidence (>32 reads; Methods) (Supplementary Data 4 ). Due to the small number of sorted cells and high variability between replicates, it was not possible to determine the significance of enrichment for each clone in the sorted populations. To assess which clones produced more L-lactate than average, we used instead the criteria that a clone had to be at least 3-times more abundant in the sorted fraction relative to the unsorted fraction. This criterium returned between 500 to 900 clones per sorted sample. Further filtering of clones enriched in at least two of the four sorted samples returned 397 clones, 266 harbored sgRNAs targeting ORFs and 131 harbored sgRNAs targeted to ncRNAs. Twenty-three clones were enriched in three of the four samples, and one clone was enriched in all four samples. 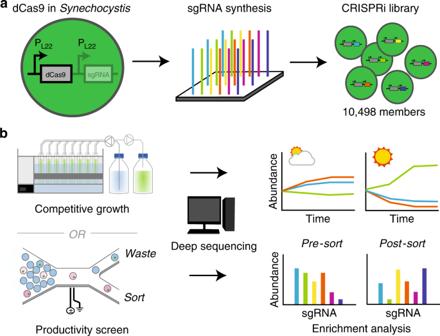Fig. 1: Workflow for CRISPRi screening inSynechocystis. aCreating the CRISPRi library. An inducible promoter PL22is used inSynechocystis.bThe fitness or productivity of each library member is assessed by counting mutants in a bioreactor cultivation or in a sorted population using next-generation sequencing. Though nearly half of the enriched clones targeted genes of unknown function, it is possible to derive engineering strategies from the annotated targets (Table 1 ). Alterations in carbon flux in cyanobacteria can be achieved by restriction of nutrient uptake or assimilation [35] , [36] , [37] . Enriched targets in nutrient uptake include glutamate dehydrogenase ( gdhA ), glutamate synthase ( gltB ), and glutamine synthase ( glnA) , repression of these would restrict NH 3 assimilation, as well as a nitrogen transporter (nrtD2 ) and a phosphorous transporter ( pstC ). Direct alteration of carbon flux was also apparent among enriched clones. For example, repression of 3-phosphoglycerate dehydrogenase ( serA ), citrate synthase ( gltA) , and phosphoketolase ( slr0453) could each be expected to increase pools of pyruvate, the precursor to L-lactate [31] , [38] , [39] . A second engineering strategy is suggested by target genes in electron transport and energy metabolism. Computational [40] , [41] and experimental [42] , [43] studies have shown that efficient production of some biochemicals would require lowering the ATP/NADPH ratio in the cyanobacteria cell. The enriched targets ssr2016 and ndhD2 are both involved in ATP-generating cyclic electron flow around PSI in Synechocystis [44] . SdhB is a subunit of succinate dehydrogenase contributing to respiration. The flavodiiron protein flv3 ( sll0550 ) catalyzes photoreduction of O 2 during stress conditions. Knockout of flv3 was shown to lower cellular ATP/NADPH ratio in Synechocystis [43] . Finally, the CCA-tRNA nucleotidyltransferase pcnB , essential for tRNA maturation and thus protein synthesis, was also enriched. Table 1 Selection of sgRNA clones enriched by droplet sorting. Full size table We reconstructed eight clones for validation of L-lactate productivity, representing targets within nutrient uptake, carbon flux, and redox and energy generation (Table 1 ). In a first screen, we cultivated clones in shake-flasks. Cultures were induced for gene repression 2 days prior to inoculation. Only the gltA and pcnB strains had a significantly higher L-lactate titer than the control strain (Fig. 6a ). The effect was enhanced when titers were normalized to cell density, indicating a redirection of carbon flux from biomass formation to product [38] . Two of the potentially redox-altered mutants ( sdhB, ssr2016 ) were tested in a photonfluxostat reactor, where light intensity was gradually increased with cell density to ensure a fixed light dosage per cell [45] . This cultivation mode was expected to activate alternative electron flow reactions for an extended time, so as to amplify any effects of repressing these on L-lactate productivity. In photonfluxostat mode, the sdhB and ssr2016 clones again had higher L-lactate titers than the control strain, but variability was high and the effect was not statistically significant (Fig. 6b ). We note that titers and specific productivities were lower for all strains in the photonfluxostat mode than in shake-flasks, which could be due to altered gas transfer or different perceived light intensities. Fig. 6: SgRNA clones with increased L-lactate production. Mutants with potentially increased L-lactate productivity were discovered using a fluorescence-activated droplet sorting assay. Seven selected mutants were reconstructed, cultivated, and product titer determined in µmol per liter, and µmol per liter per biomass (OD 720 nm ). a Productivity of selected mutants cultivated in axenic shake-flask cultures (n = 2, each strain assayed in two independent replicates). L-lactate concentration was measured after 24 and 48 h. NT0 - control sgRNA with no target site in Synechocystis genome. *—significant with p ≤ 0.05, two-sided student’s t -test, pcnB, p = 0.016, gltA, p = 0.021. Bars are average values and individual values are shown as points. b A subset of two mutants was cultivated in axenic ‘photonfluxostat’ cultures (light intensity proportional to cell density, 1000 µmol photons m −2 s −1 OD 720 nm −1 , n = 2, each strain assayed in 2 separate experiments). L-lactate concentration was measured after 18 and 30 h. Bars are average values and individual values are shown as points. Source data are provided as a Source Data file. Full size image We have primarily used the CRISPRi repression library to identify potential mutants with improved industrial phenotypes, which we then validated with screening of individual clones. By providing fitness contributions of all genes in a certain condition, the CRISPRi library reveals patterns in how cyanobacteria could solve certain physiological challenges. There were multiple genetic avenues for enhancing the growth rate of Synechocystis , though they converged on a similar transcriptome that upregulates photoprotection and electron-transport around PSI. An increase in PSI activity at high light can dissipate pressure in the electron-transport chain; a similar phenomenon was reported to contribute to high-light tolerance and faster growth in Synechococcus elongatus UTEX 2973 compared to its close relative Synechococcus PCC 7942 [46] . This is also in-line with a recent modeling study, which showed that the rate of ATP and NADPH generation exerted the most control over carbon fixation rates in Synechocystis [47] . Interestingly, four out of five sgRNA targets in top faster-growing strains are potentially regulator proteins ( pmgA , slr1916 , ssl2982 , slr1340 ). This finding is reminiscent of the mutation in the master regulator RpaA of Synechococcus elongatus UTEX 2973 that drastically alters the transcriptome and is necessary for unlocking fast growth [48] . The RNAP omega subunit ( ssl2982 ) is critical for acclimation of Synechocystis from low to high CO 2 [49] . That repression of ssl2982 provides a growth advantage at high light and high CO 2 is surprising. However, our experimental setup differs from that used previously, in that we perform a knockdown of ssl2982 , and that cells are already pre-acclimated to high CO 2 before repression. Care should be taken when using results from CRISPRi libraries to determine gene essentiality. We used 2 sgRNAs targeting each ORF; recent studies have shown that more are needed to ensure statistical significance when assessing gene essentiality [12] . Furthermore, a confident determination of gene essentiality from CRISPRi data would require consideration of a gene’s place in an operon. Data from an E. coli CRISPRi library showed a strong polar effect, where targeting the first gene in an operon also represses downstream genes, while the reverse polar effect, i.e., repression of downstream genes affecting expression of upstream genes, was not prominent [50] . For Synechocystis , transcription start sites have been mapped in detail for several growth conditions and are annotated in the reference genome ( NC_000911.1 ) [15] . Therefore, fitness data for individual genes can be considered with their operon context. For example, the pyk2 gene (sll1275) encoding pyruvate kinase 2 is at the 5′ end of an operon that also contains sll1276 (probable iron transporter) and recF downstream. In our data, both sgRNA clones targeting pyk2 showed severe growth defects, suggesting it is important for cell growth. However, one sgRNA clone targeting sll1276 also shows a strong growth defect. Considering previous attempts to knockout sll1276 were unsuccessful [51] , it is likely that sll1276 is essential for cell growth. Based on the sgRNA data alone, we cannot unambiguously conclude that pyk2 is essential for growth, as the downstream sll1276 is also likely repressed in those clones. For ~50% of the genes with low fitness scores in our data, one sgRNA was significantly depleted from the library and the other was not (Supplementary Fig. 11 ). There are several lines of evidence which suggest that this discrepancy is due to weak binding of one of the sgRNAs (a false-negative) instead of off-target binding of an sgRNA to an essential gene elsewhere (false-positive). First, while repression efficiency of sgRNAs targeting near the start codon is typically >90%, it can be as low as 50%, so partial repression of an essential gene may not elicit a phenotype [13] . Second, 86% (283/329) of genes predicted to be essential by Flux Balance Analysis of a Synechocystis genome-scale model had at least one associated sgRNA clone significantly depleted [52] (p adj < 0.005; Supplementary Data 5 ). There is also a 75% agreement in our calculated fitness scores for genes in central carbon metabolism to their orthologs in Synechococcus PCC 7942, the latter determined by Tn-Seq [8] (Supplementary Data 6 ). Third, off-target binding by dCas9 was shown to be problematic for strongly expressed dCas9 [50] , while our genome-integrated dCas9 was driven by a weak promoter. However, dCas9 is potent, as we observed gene repression for some targets even in the absence of the inducer (Cluster 1 in Fig. 2 ). Finely-graded dCas9 expression may require native, metal-sensitive promoters [53] , or addition of translational-level control such as riboswitches [54] . The CRISPRi library has a unique advantage over gene knockouts for engineering bioproduction in that the level of essential genes can be titrated, allowing perturbation of the core metabolic network [55] . Cultures where a ‘metabolic switch’ shifts metabolism away from growth can be more productive [14] , [38] , [56] , [57] . By coupling the CRISPRi library to a fluorescence assay, we were able to screen thousands of potential knockdowns for increased productivity, giving a test of many metabolic engineering strategies previously proposed by computational modeling. However, several limitations were apparent in the library-droplet microfluidics workflow. CRISPRi induction must be optimally timed before sorting. The 4 h incubation period where cells secrete L-lactate generates high single-cell variability and is dependent on cell shading, though we attempted to counter this with a high screening depth. This short incubation period was necessary to prevent saturation of the fluorescence assay. Larger droplet sizes would allow for longer incubation times. In batch validation, not all of the enriched clones from the droplet sorting gave higher L-lactate titer and there were apparent tradeoffs between productivity and carbon partitioning in some clones. Therefore, we propose that the CRISPRi library is most useful for revealing principles for guiding engineering, and that clones must be validated. It is easy to envision expanding an inducible CRISPRi library to other screens. Strains with faster growth rate may not be robust under stress conditions. For example, the pmgA and slr1916 mutants grew faster than the control strain in L100, L300, and LD conditions, but slower under lactate stress. Further, pmgA and slr1916 knockout strains are known to be glucose sensitive in the light, as photosystem stoichiometry cannot adapt to additional reductant supply from sugar metabolism [21] , [22] . Repression of ssl2982 increases growth in L300 condition, but a knockout mutant is known to be sensitive to shifts in CO 2 and temperature [58] . Challenging the CRISPRi library to fluctuating conditions would allow a deeper study of the tradeoff between growth speed and robustness. Since the two fastest-growing mutants found here were also glucose sensitive, it could be worthwhile to add a screen for photomixotrophic growth, which results in flux through alternative glycolytic pathways [59] . Small transposon libraries (300 mutants) have previously been used to identify genes required for phototaxis by screening for colony smearing; [60] a CRISPRi library could accelerate identification of genes involved in motility. A fluorescence-activated cell sorting (FACS) screen for cell fluorescence could be useful in mapping the photobleaching program during nutrient limitation and screens for recovery ability from starvation could identify carbon metabolism pathways involved in resuscitation [52] . Finally, libraries limited to a subset of target genes would be amenable to multiplexing of gene repression [61] . Genetic constructs and cloning of sgRNA library A catalytically dead Cas9 (dCas9, mutations D10A and H840A) from Streptococcus pyogenes was used for gene repression in this study and the Synechocystis base strain containing the tetR _P L22 _ dCas9 expression cassette in the psbA1 locus (spectinomycin resistance) [13] . The sgRNA library oligos were synthesized on a 12 K chip by CustomArray Inc., USA (see Supplementary Data 1 for a list of all sgRNA sequences). Plasmid pMD19-T (Takara) was used to create the sgRNA library. First, the homology region around locus slr0397 , the PL22_sgRNA-NT0 expression cassette, and a kanamycin resistance gene were cloned into pMD19-T by BioBrick assembly. The sgRNA library oligos were then cloned into this vector using Golden Gate assembly. NEB 10-beta Competent E. coli cells (New England BioLabs) were used for transformation and ~1,200,000 E. coli colonies were obtained. All colonies were collected, resuspended in LB, pooled together, and then cultivated overnight in LB. The plasmid DNA was extracted using the ThermoFisher Maxi plasmid extraction kit. Natural transformation was used to transform the plasmid (10 μg) in Synechocystis [62] , where ~300,000 colonies were obtained. Colonies were collected, resuspended in fresh BG-11 and pooled. The pooled Synechocystis library was stored at −80 °C. To re-create specific sgRNAs for clone validation, we used overlap-extension PCR of a template sgRNA to introduce the protospacer [13] . All primers are listed in Supplementary Data 7 . The L-lactate-secreting Synechocystis strain was created by cloning the ldh gene with L39R substitution from Lactococcus lactis under the P trc promoter [32] . This gene construct was inserted into the genome at locus slr0168 with a chloramphenicol resistance cassette. This strain was subsequently transformed with the tetR _P L22 _ dCas9 cassette and sgRNA library as described above, resulting in a L-lactate-producing Synechocystis sgRNA library. All strains and plasmids are available from the authors upon request. sgRNA library design Two sgRNAs were designed for each open reading frame (ORF) and non-coding RNA in the Synechocystis genome (Reference genome NCBI NC_000911.1, [ https://www.ncbi.nlm.nih.gov/nuccore/NC_000911.1 ]). ORF sequence annotations were obtained from NCBI (downloaded on 18.03.2016). Locations of non-coding RNAs were from Kopf and Hess [15] , [63] . An in-house Python script was used to create protospacer sequences as close to the transcription start site (TSS) or translation start codon (ATG) as possible, within the following criteria: Target regions were required to be within 500 bp from the known TSS or within 75% of total gene length, absence of G 6 and T 4 , and GC content between 25 and 75%. Target sequences were searched according to the pattern 5′-CCN[20-25 bases]T-3′. The 5′-CCN ensured a 5′-NGG-3′ PAM site on the coding strand, and 3′ T was to ensure binding of the 5′ end of the sgRNA, known to have an A when transcribed from promoter P L22 in Synechocystis [64] . For each target fitting these criteria, potential off-target regions in the genome were then identified. An off-target binding site defined as having fewer than two mismatches in the PAM-proximal 17 bp region of the proposed sgRNA. Both NGG and NAG PAMs and both strands were considered. Then all sgRNA candidates for a gene, the two sgRNAs with the least off-targets were selected. If possible, sgRNAs were selected that were at least 10 bp apart from each other. The in-house Python script is publicly available at [ https://github.com/KiyanShabestary/2019_CRISPRi_library ]. Cultivation in photobioreactor turbidostats The Synechocystis sgRNA library was cultivated in an 8-tube photobioreactor (Multi-Cultivator MC-1000-OD, Photon System Instruments, Drasov, CZ). The system was customized to perform turbidostat cultivation [16] . Reactors (65 mL) were bubbled with 1% v/v CO 2 in air (2.5 mL/min) at 30 °C, and light intensity was controlled by a computer program. The OD 720 nm and OD 680 nm were measured every 15 min. The turbidity set point was OD 720 nm = 0.2 and 22 mL fresh BG-11 was added to dilute the culture once the set point was exceeded. Antibiotics (25 µg/mL spectinomycin, 25 µg/mL kanamycin) and anhydrotetracycline inducer (500 ng/mL) was added to the culture and the reserve BG-11 media used for dilution. For LD cultures, the light regime (12 h light − 12 h dark) followed a sinusoidal function with maximum light intensity at 300 µmol m −2 s −1 (L (t) = 300 ∗ sin (π/43200 ∗ t) where t = cultivation time in seconds). For turbidostat cultivations with added L-lactate, light intensity was 100 µmol m −2 s −1 and either 100 mM sodium L-lactate or 100 mM NaCl was added to the BG-11 before inoculation and medium pH was adjusted to 7.8. All turbidostat cultivations described in this work were performed as four independent replicates. To sample for NGS, 15 mL of culture volume was harvested by centrifugation (5,000 × g for 5 min, 25 °C). Cells were collected and stored at −20 °C. Batch cultivations for growth rate or L-lactate quantification of selected sgRNA mutants were performed in the same conditions as turbidostat cultures, but with light at 300 µmol photons m −2 s −1 . Mutants were pre-cultivated in BG-11 with antibiotics (25 µg/mL spectinomycin, 25 µg/mL kanamycin) and aTc inducer (added to 500 ng/mL) in a climatic chamber (Percival Climatics SE-1100 with 100 μE/s/m 2 illumination,1% v/v CO 2 at 30 °C) for 3 days, and then inoculated into the photobioreactor to OD 730 nm = 0.05 before growth measurements began. Next-generation sequencing of sgRNA region A two-step PCR procedure was carried out for NGS library preparation using sgRNA library plasmid from E.coli or genomic DNA from Synechocystis library as template. Genomic DNA was extracted from Synechocystis cell pellets (15 mL culture at OD 720 nm 0.2) using GeneJET Genomic DNA Purification Kit (Thermo Fisher Scientific). 1st step PCR was performed using the primer pair LUYA593/LUYA594, which amplify sgRNAs from the plasmid or genome and add adaptors for NGS. The PCR product was analyzed on Agilent 2100 Bioanalyzer (Agilent Technologies) and gel purified using GeneJET Gel Extraction Kit (Thermo Fisher Scientific). The purified DNA was used as template to perform the 2nd step PCR using NEBNext Multiplex Oligos for Illumina (Dual Index Primers Set 1) (New England Biolabs), followed by Bioanalyzer analysis and gel purification. Purified DNA was quantified using Qubit fluorometer 2.0 (Thermo Fisher Scientific) and then pooled. The NGS was performed on Illumina NextSeq 500 system using NextSeq 500/550 High Output v2 kit (75 cycles). In a typical NGS run, 40 samples were analyzed simultaneously, providing 50–100 reads per sgRNA per sample (Supplementary Fig. 12 ). We used sickle 1.33 [ https://github.com/najoshi/sickle ] to trim (75 nt) and clean reads. A custom python script was used to assign and count reads to each sgRNA, available at [ https://github.com/KiyanShabestary/2019_CRISPRi_library ]. Fitness score calculation The gradual, sgRNA-mediated depletion of clones from the library allows estimation of the contribution to cellular fitness for each individual gene. Here, we defined the fitness F of a mutant as the area under the curve (AUC) for log 2 fold-change sgRNA abundance (log 2 FC) at a number of generations (n gen ) since induction, normalized by maximum generations. F = AUC( n_gen,log_2FC)/maximum(n_gen)
 (1) 
    Δ F = F_L300 - F_L100
 (2) Differential fitness Δ F between two conditions, e.g., L300 and L100, was calculated according to Eqs. 1 and 2 . RNA extraction and sequencing Synechocystis fast growing mutant strains as well as the control strain (sgRNA-NT0) were cultivated in photobioreactor in turbidostat mode under the same conditions as they were enriched (see above). At 3 days post induction, 40 mL culture (OD 730 nm = 0.2) was sampled. Cells were collected by centrifugation for 5 min at 4 °C, and total RNA was extracted immediately afterwards. Ribosomal rRNA was depleted using Illumina Ribo-Zero rRNA Removal Kit (Bacteria). Library preparation was carried out using NEBNext Ultra II Directional RNA Library Prep Kit (New England Biolabs) following manufacturers guidelines. Libraries were sequenced on Illumina NextSeq 500 System using NextSeq 500/550 High Output v2 kit (75 cycles). RNA sequencing reads were filtered and mapped to the genome using Ribopipe [65] . Filtering entailed adapter removal with cutadapt 1.18, quality trimming with sickle 1.33, and rRNA and tRNA removal using Bowtie 1.2.2 and reference sequences from the Synechocystis genome (Reference genome NCBI NC_000911.1, [ https://www.ncbi.nlm.nih.gov/nuccore/NC_000911.1] ). Bowtie v. 1.2.2 was used to map the filtered reads to the Synechocystis genome. The number of reads mapping to each gene in each sample was counted and formatted using custom Python and R scripts available at [ https://github.com/Asplund-Samuelsson/ribopipe ]. RNA sequencing data were initially processed as described before for NGS sequencing of library data. DESeq2 was used to determine fold changes between conditions as well as significance (three independent biological replicates). Significant genes were selected based on the following two criteria: absolute log 2 FC ≥ 1, adjusted p -value ≤ 0.05). Unsupervised clustering of significantly different genes based on expression in all mutants was performed as described for NGS data analysis. Statistical analysis of library competition data All analyses were performed using the R programming language and are documented in R markdown notebooks available at [ https://m-jahn.github.io/ ]. Data for all competition experiments performed with the sgRNA library can be accessed at [ https://m-jahn.shinyapps.io/ShinyLib/ ]. First, data tables from different sequencing runs were merged into a single master table. For simplicity, harvesting time-points 12 and 30 days for the sodium chloride condition (NACL) were re-labelled as 16 and 32 days to correspond to time-points of all other samples. This did not influence the calculation of generation time or fitness score, and was done only to display these samples along with corresponding L-lactate samples. The R package DESeq2 was used to determine fold changes between conditions as well as significance metrics (multiple hypothesis adjusted p -value, Benjamini-Hochberg procedure) [66] . Fold changes and p -values were determined using four independent biological replicates for all cultivations. Gene-wise annotation was added based on Uniprot (IDs, protein properties, GO terms) and CyanoBase (functional categories). 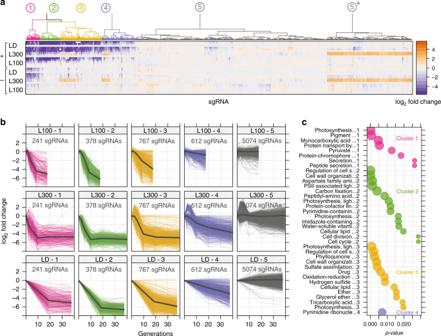Fig. 2: Dynamics of CRISPRi library during photoautotrophic growth. aClustered sgRNAs by similarity of log2fold-change over time. Rows represent time-points sampled after induction. (L100—light with 100 µmol m−2s−1, L300—light with 300 µmol m−2s−1, LD—light-dark cycle). All log2fold-change values were calculated from averages of four replicate cultivations. Symbols: plus, induced, minus, non-induced, star, cluster 5 is a combination of two unchanged clusters.bLog2fold-change of individual sgRNAs over the course of each cultivation. Experiment run time was normalized to number of cell generations estimated from population growth rate.cEnriched gene-ontology (GO) terms for the four clusters (1–4) showing sgRNA depletion;p-value—Fisher’s exact test with elimination (see Methods). Source data are provided as a Source Data file. Altogether 7119 unique sgRNAs corresponding to 3541 unique genes (without non-coding RNAs) were included in the analysis. The coverage per sample in terms of quantified sgRNAs and median read count per gene is shown in Supplementary Fig. 12 . Unsupervised clustering of sgRNA data To cluster sgRNAs based on depletion/enrichment pattern, a dissimilarity matrix was computed using R’s dist function with distance measure euclidean. Clustering was performed using function hclust with method ward.D2. Silhouette analysis was performed to find the optimal number of clusters (silhouetteAnalysis from package silhouette) and showed equally good separation for 3–9 clusters. A number of six clusters was chosen representing sgRNAs with decreasing level of depletion (1–4) as well as two clusters with unchanged sgRNAs (5 and 6). These two clusters were separated by a group of sgRNAs (around 25% of all) that showed a spurious, temporary enrichment for two specific time-points (1 and 2 day measurements). This temporary enrichment was most likely due to technical variation (e.g., in sample preparation) and has no biological explanation. Clusters 5 and 6 were therefore combined in cluster 5 (Fig. 2a ). Gene-ontology enrichment For gene-ontology (GO) term enrichment, the TopGO package by Alexa et al. was used to determine GO terms associated with sgRNAs for clusters 1–4 (TopGO method ‘Fisher, eliminating’) [67] . The resulting list of GO terms was filtered by dispensability scores obtained using REVIGO ( http://revigo.irb.hr/ , threshold ≤ 0.5). Furthermore, GO terms annotated with less than 5 or more than 200 unique sgRNA/genes or p -value > 0.03 were filtered out. Enrichment of sgRNA mutants with increased L-lactate tolerance To find genes involved in L-lactate tolerance, sgRNAs enriched specifically for presence of sodium L-lactate but not sodium chloride were selected (threshold: log 2 FC ≥ 2, −log 10 p -value ≥ 20). Twenty-four and 75 sgRNAs were found to be enriched after 16 and 32 days, respectively (Fig. 5a ). The 24 sgRNAs enriched after 16 days were included in the set of 75 sgRNAs enriched after 32 days. In contrast to the 75 sgRNAs that were enriched, thousands of sgRNAs were depleted during growth in the presence of L-lactate. To find sgRNAs specifically depleted under L-lactate but not sodium chloride, a differential fitness score was calculated between the two conditions ( dF = F NaCl − F Lac ). 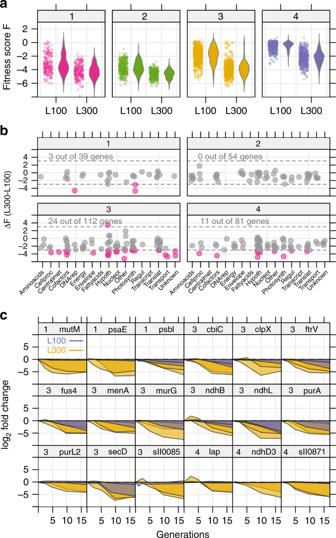Fig. 3: Genes with condition-dependent fitness in two light conditions. aDistribution of fitness scoreFfor all sgRNAs in clusters 1–4 (color code as in Fig.2). Fitness score indicates the degree of enrichment (positive) or depletion (negative) of an sgRNA, normalized to cell generations. Comparison between two light conditions (L100—light with 100 µmol m−2s−1and L300—light with 300 µmol m−2s−1) shows sgRNAs are on average more rapidly depleted under L300 independent of number of cell generations.bDifference in fitness (ΔF) between L100 and L300, for genes with both sgRNAs in the same cluster. Differentially depleted/enriched sgRNAs indicated in red, threshold: 3 ≤ ΔF ≤ −3.cTime courses of both sgRNAs for a selection of 18 genes with high ΔFin L100 (blue) and L300 (yellow). Source data are provided as a Source Data file. The top 200 sgRNAs with highest dF were selected and six genes were found with both sgRNAs strongly depleted (see also Supplementary Fig. 9 ). Estimation of mutant growth rates The change in a mutant’s abundance within the total population, combined with the population average growth rate (known from the dilution rate of the turbidostat), allows estimation of the growth rate of each mutant. The rate of enrichment or depletion of a mutant ( μ diff ) was defined as the population growth rate ( μ pop ) subtracted by the mutant’s individual growth rate ( μ mut ) (Eq. 3 ). μ_diff = μ_pop - μ_mut
 (3) The depletion of a mutant from the library can be modeled as a function of time, where the mutant fraction f at time point t becomes: 
    f(t) = f(t = 0) ×( 1 - (μ_pop - μ_mut))^t
 (4) The mutant fraction f at different times and the average growth rate of the population are known parameters, allowing to estimate growth rate for all mutants (Eq. 4 ). Correlation between gene expression variability and fitness To correlate gene fitness (obtained from sgRNA library competition experiments) with variability in gene expression, the proteomics dataset PRIDE PXD009582 was used [16] . The dataset contains mass spectrometry based protein measurements of Synechocystis for 2000 proteins at five different growth rates, each for CO 2 and light limitation. The variability of a protein was defined as growth-rate dependent change in abundance, and determined as p -value from analysis of variance (ANOVA). If a protein changed abundance significantly with growth rate (either up or downregulation) a lower p -value was obtained. Proteins were binned into groups according to p -value ranges (1–0.1, 0.1–0.05, 0.05–0.01, 0.01–0.001, <0.001) and fitness score of sgRNAs associated with the respective proteins in a group were plotted. Absorption spectrum of L-lactate-tolerant mutants Selected mutants as well as the control strain (sgRNA-NT0) were cultivated in 30 mL BG-11 supplemented with 100 mM sodium L-lactate in shaking flasks at 100 µmol photons m −2 s −1 continuous light, and 500 ng/mL aTc was added at the beginning of the cultivation. 0.5 mL cell culture was sampled after induction for 3 days and cells were collected by centrifugation at 5000 × g for 10 min. Cells were then washed twice with 1 mL PBS by centrifugation and resuspension, and then resuspended in 400 µL PBS. Two times 100 µL resuspended cells were transferred to a transparent 96-well plate. Absorption spectra of cell samples were obtained in the range of 350–800 nm using a photospectrometer (SpectraMax M5, Molecular Devices). Absorption spectra were normalized to the reference A 720 nm and relative chlorophyll a, phycocyanin and carotenoid content of cells were determined using the ratio of A 680 nm /A 720 nm , A 630 nm /A 720 nm , and A 490 nm /A 720 nm , respectively. Droplet microfluidic screening of L-lactate-producing sgRNA library The L-lactate-producing Synechocystis sgRNA library was grown in shake-flasks in a climatic chamber. Cultures were supplemented with antibiotics (12.5 µg/mL chloramphenicol, 25 µg/mL spectinomycin) and aTc (1 μg/mL). For the productivity assay, cells were harvested (OD 720 nm = 0.4-0.6), washed to OD 720 nm = 0.15, and encapsulated into droplets [68] . A mix of HFE-7500 oil and 1% (w/w) EA surfactant droplet stabilizer (RainDance Technologies) was loaded into a Gastight 5-mL glass syringe (Hamilton). Cells were encapsulated in 10 pL droplets using a flow rate of 400 μL/h for the aqueous solution and 2000 μL/h for the oil. The emulsion was collected in a 1-mL plastic syringe at a withdrawal flow rate of 2000 μL/h. The syringes were connected to the chip by polyether ether ketone tubing, and flow rates were controlled by neMESYS syringe pumps (Cetoni GmbH). The droplet emulsion was incubated in an illuminated syringe (approximately 150 μE/s/m 2 ) for 4 h for L-lactate secretion. Three pL of a fluorescence-based L-lactate assay mixture (Cayman Chemical) was then injected into each droplet using a picoinjection chip [69] . The emulsion was injected at a flow rate of 70 μL/h, spacer oil separated the droplets at a flow rate of 500 μL/h and the lactate assay mixture was injected at 30 μL/h. The picoinjected emulsion was collected in a 1 mL plastic syringe protected from light. After 40 min of picoinjection, the collected emulsion was gently mixed and re-injected into a droplet sorting device(Supplementary Fig. 9 ). The flow rates used were 1000 µL/h for the spacer oil and side oil, and the emulsion was injected at 100 µL/h, corresponding to a droplet sorting rate of 1.5 kHz. Sorted droplets were collected using a withdrawal rate of 1000 µL/h. Approximately 1,800,000 droplets were screened and the top 2% most fluorescent droplets were sorted, corresponding to approximately 36,000 droplets. 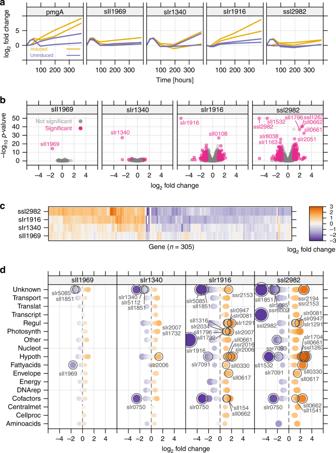Fig. 4: Transcriptomics of faster-growing mutants. aEnrichment of faster-growing sgRNA mutants in library competition (turbidostat) experiment at L300 (300 µmol photons m−2s−1), log2fold-change of read count over time (n= 2 sgRNAs).bVolcano plot representation of transcriptomics data from four reconstructed sgRNA mutants. Shows log2fold-change for gene expression compared to the control strain (sgRNA-NT0), against adjustedp-value for each gene. Gray—non-significantly different genes, pink—significantly different genes (threshold: negative log10p-value ≥ 2; absolute log2fold-change ≥ 1). Thep-value for three sgRNA mutants was outside the plotting region and was restricted to −log10of 50 for visibility.cHeat map representation of transcriptomics data from four reconstructed sgRNA mutants. Shows all 305 genes that were significantly different in at least one of the four mutants, clustered into two different groups based on similarity of gene expression.dSignificantly different genes are sorted by Cyanobase pathways. Genes of particular interest were highlighted (see text for details). Blue and orange indicates negative and positive log2fold-change, respectively. Size of symbols increases with increasing absolute change. Source data underlying Fig.4b, dare provided as a Source Data file. After sorting, the collected emulsion was broken with 10% v/v 1 H, 1 H, 2 H, 2H-perfluoro-1-octanol (Sigma Aldrich), followed by centrifugation and evaporation to remove the residual liquid. Cells were resuspended in DMSO and heated at 95 °C for 2 min to release genomic content. 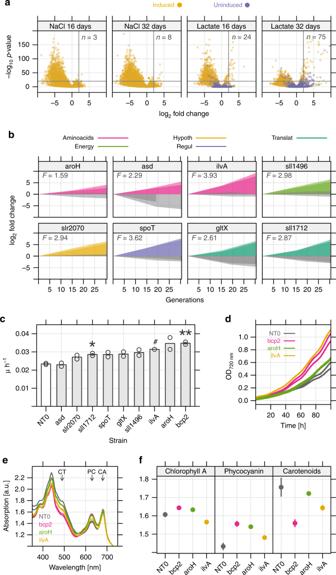Fig. 5: SgRNA clones with improved L-lactate tolerance. aVolcano plot showing enrichment of 75 sgRNAs during cultivation with added 0.1 M sodium L-lactate after 32 d, (threshold: log2fold-change ≥ 2, −log10p-value ≥ 20). Only 8 sgRNAs were enriched in a 0.1 M NaCl control cultivation.bEight genes where both sgRNAs were enriched above average in 0.1 M L-lactate cultivation (coloured) but not NaCl cultivation (gray). Color indicates association to a cyanobase pathway.F- mean fitness score of two sgRNAs.cMean growth rate µ (h−1) of selected, reconstructed knockdown strains (n= 2 independent replicate cultivations) over the first 80 h of batch cultivation with L-lactate added to 0.1 M. Symbols show significance between the control strain (NT0) and mutants using 1-sided student’st-test. *p-value ≤ 0.05, **p-value ≤ 0.01 (sll1712,p= 0.019; bcp2,p= 0.006), #—only 1 replicate was used forilvAmutant.dExample of growth advantage in batch culture with L-lactate added to 0.1 M of sgRNA clonesbcp2,aroH, andilvA.eAbsorption spectra of fastest-growing sgRNA mutants and NT0 in 0.1 M L-lactate. Arrows mark absorption maxima for pigments. CT carotenoids, PC phycocyanin, CA chlorophyll A.fRelative pigment absorption for carotenoids, phycocyanin, and chlorophyll A for the selected strains with L-lactate added to 0.1 M. Source data underlying Fig.5a, bare provided as a Source Data file. 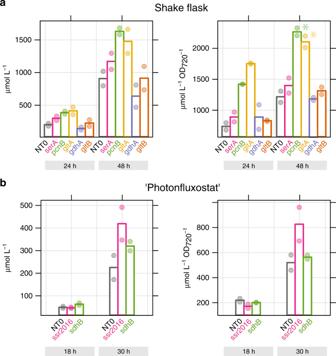Fig. 6: SgRNA clones with increased L-lactate production. Mutants with potentially increased L-lactate productivity were discovered using a fluorescence-activated droplet sorting assay. Seven selected mutants were reconstructed, cultivated, and product titer determined in µmol per liter, and µmol per liter per biomass (OD720 nm).aProductivity of selected mutants cultivated in axenic shake-flask cultures (n = 2, each strain assayed in two independent replicates). L-lactate concentration was measured after 24 and 48 h. NT0 - control sgRNA with no target site inSynechocystisgenome. *—significant withp≤ 0.05, two-sided student’st-test, pcnB,p= 0.016, gltA,p= 0.021. Bars are average values and individual values are shown as points.bA subset of two mutants was cultivated in axenic ‘photonfluxostat’ cultures (light intensity proportional to cell density, 1000 µmol photons m−2s−1OD720 nm−1,n= 2, each strain assayed in 2 separate experiments). L-lactate concentration was measured after 18 and 30 h. Bars are average values and individual values are shown as points. Source data are provided as a Source Data file. The cell lysate was used as template to directly amplify the sgRNA region using primer pair LUYA271/LUYA300. Then adaptors were incorporated into the PCR product using primer pair LUYA593/LUYA594, followed by NGS library preparation as described above. Droplet microfluidics NGS data filtering Using NGS obtained on each sorted droplet fraction, we could map 5 million reads per sample, covering to 8000–10,000 unique sgRNAs. sgRNAs with fewer than 32 mapped reads in a sample were removed from that sample. To calculate ‘enrichment factors’ for each sgRNA, the relative abundance of the sgRNA in the sorted droplet was divided by its relative abundance in the total library before droplet encapsulation. Next, sgRNAs where the enrichment factor differed ≥10-fold between replicates were removed. The remaining sgRNAs were then ranked by enrichment factor for each sorted sample. sgRNAs at least three times more abundant in sorted fraction relative to unsorted fraction were given a score of 1 for that sample. Clones with a score 2/4, summed over all samples were determined to have potential to increase L-lactate productivity. L-lactate production in batch and photonfluxostat The L-lactate-producing Synechocystis sgRNA library mutants were first cultivated in shake-flasks in a climatic chamber. Cultures were pre-cultivated in BG-11 supplemented with antibiotics (12.5 µg/mL chloramphenicol, 25 µg/mL kanamycin) and induced with aTc (1 μg/mL) 2 days prior to the start of the experiment. Then mutants were transferred to shake-flasks or in an 8-tube photobioreactor (see library cultivation methods) with a starting OD 720 nm of 0.1, supplemented with aTc and antibiotics as stated above. Cultures in the photobioreactor were grown in a ‘photonfluxostat’ mode, where light is increased based on cellular density to extend log phase. The amount of light given to the culture is equal to the cellular density multiplied by a light regime factor (1000 µmol photons m −2 s −1 OD 720 nm −1 ). L-lactate was measured using a L-lactate fluorescent kit (Cayman Chemical) according to the manufacturer’s instructions. Reporting summary Further information on research design is available in the Nature Research Reporting Summary linked to this article.